Cellular protection using Flt3 and PI3Kα inhibitors demonstrates multiple mechanisms of oxidative glutamate toxicity Glutamate-induced oxidative stress is a major contributor to neurodegenerative diseases. Here, we identify small-molecule inhibitors of this process. We screen a kinase inhibitor library on neuronal cells and identify Flt3 and PI3Kα inhibitors as potent protectors against glutamate toxicity. Both inhibitors prevented reactive oxygen species (ROS) generation, mitochondrial hyperpolarization and lipid peroxidation in neuronal cells, but they do so by distinct molecular mechanisms. The PI3Kα inhibitor protects cells by inducing partial restoration of depleted glutathione levels and accumulation of intracellular amino acids, whereas the Flt3 inhibitor prevents lipid peroxidation, a key mechanism of glutamate-mediated toxicity. We also demonstrate that glutamate toxicity involves a combination of ferroptosis, necrosis and AIF-dependent apoptosis. We confirm the protective effect by using multiple inhibitors of these kinases and multiple cell types. Our results not only identify compounds that protect against glutamate-stimulated oxidative stress, but also provide new insights into the mechanisms of glutamate toxicity in neurons. Oxidative stress is implicated in a number of neurological diseases, including ischaemic stroke, amyotrophic lateral sclerosis, Parkinson’s disease and Alzheimer’s disease [1] , [2] . Glutamate toxicity is a commonly used model to study oxidative stress-induced neuronal cell death associated with both acute and chronic neurological insults [2] . In this model, neuronal cells are incubated with high concentrations of extracellular glutamate, which inhibits cystine uptake into the cells via the cystine/glutamate antiporter, leading to glutathione (GSH) depletion and accumulation of reactive oxygen species (ROS) [3] , [4] , [5] . Although the increase in intracellular ROS caused by GSH depletion mediates oxidative glutamate toxicity (oxytosis), it is not the only mechanism of glutamate-induced neuronal cell death [5] , [6] . For example, caspase-independent apoptotic pathways involving activation of 12-lipoxygenase and subsequent translocation of apoptosis-inducing factor (AIF) have also been implicated [7] , [8] . In addition, ferroptosis is a recently described form of cell death, which may be involved in glutamate toxicity in neurons, as shown by a recent study in which inhibition of ferroptosis prevented glutamate-induced cell death in organotypic hippocampal slice cultures [9] . Nevertheless, whether glutamate toxicity occurs via apoptosis, necrosis, ferroptosis or another form of cell death is a subject of some controversy, and our understanding of the molecular mechanisms underlying glutamate oxytosis is still incomplete [10] . Therefore, elucidation of the pathways leading to neuronal cell death or survival after exposure to oxidative stress remains a critical area of research, particularly for the development of novel and effective treatments for neurodegenerative diseases. Protein kinases are major regulators of numerous key cellular pathways, including the signalling cascades that control cell survival and proliferation. In an effort to identify kinases involved in glutamate-mediated oxidative stress, we screened a kinase inhibitor library for the ability to protect neuronal cells from oxidative stress-induced cell death. Here, we show that the receptor tyrosine kinase Flt3 and the signalling molecule phosphoinositide 3-kinase α (PI3Kα) have key roles in glutamate oxidative stress-induced cell death in multiple neuronal cell lines and primary cerebrocortical neurons. We used a 1 H-nuclear magnetic resonance ( 1 H-NMR) metabolomics approach to characterize the molecular processes involved in the cell stress response and induction of death, and found that inhibitors of Flt3 and PI3Kα protected against glutamate toxicity via two distinct pathways. The PI3Kα inhibitor prevented early necrotic cell death by partially restoring intracellular levels of GSH, whereas the Flt3 inhibitor reduced both necrotic and AIF-dependent apoptotic cell death by directly preventing oxidation of polyunsaturated fatty acids (PUFAs). We also report that glutamate toxicity shares some phenotypic features with ferroptosis, including increased ROS production, a dependency on iron and involvement of PUFA metabolism. Notably, Flt3 and PI3Kα inhibitors blocked ferroptotic cell death in neurons. Collectively, the results of this study demonstrate that Flt3 and PI3Kα inhibitors are potent protectors against oxidative neuronal injury and provide new insights into the death mechanisms triggered by oxidative glutamate toxicity. Flt3 and PI3Kα are involved in oxidative glutamate toxicity We screened a kinase inhibitor library for compounds that protect neuronal cells against hypoxia (0.1% oxygen)-induced death or growth arrest in the HT22 cell line. HT22 is a mouse hippocampal cell line that lacks ionotropic glutamate receptors, resulting in glutamate-induced cell death mediated solely by oxytosis [11] . This cell line is therefore an excellent model for the study of glutamate oxidative toxicity. Our initial screen employed hypoxia as the oxidative stress inducer because we were interested in kinases involved in oxidative stress-associated glutamate toxicity. These two processes are linked by the generation of ROS [2] , [12] . Among the 244 kinase inhibitors screened, we identified nine that inhibited 0.1% hypoxia-induced cell death by at least 30%, the cut-off value for compound selection ( Supplementary Fig. 1a and Supplementary Data 1 ). The protective effects of the nine inhibitors were then confirmed in full dose-response experiments ( Supplementary Fig. 1b ). To determine whether these compounds also protected against glutamate-induced toxicity, HT22 cells were incubated with 5 mM glutamate for 18 h in the presence or absence of varying doses of inhibitors. 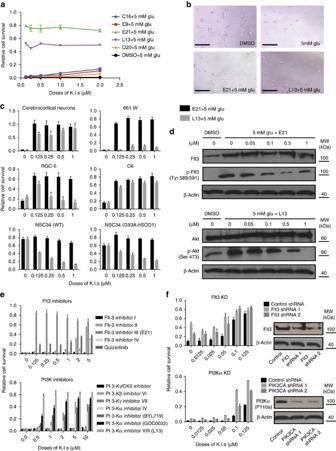Figure 1: Kinase inhibitors prevent glutamate-induced cell death. (a) Relative HT22 cell survival after treatment with 5 mM glutamate (glu) for 18 h in the presence or absence of the indicated kinase inhibitors (K.I.; seeSupplementary Table 1). (b) Phase contrast images of HT22 cells treated with 0.5 μM E21 or L13 and 5 mM glu (Scale bar, 50μm). (c) Relative cell survival of primary neurons and various neuronal cell lines treated for 18 h with the indicated concentrations of E21 or L13 in the presence of glu at: 5 mM (cerebrocortical neurons, 661W), 10 mM (NSC34) or 20 mM (RGC-5, C6). (d) Representative western blots of Flt3, phospho-Flt3, Akt, phospho-Akt and β-actin (control) in lysates of HT22 cells treated with 5 mM glu for 6 h and the indicated concentrations of E21 and L13. (e) Relative survival of HT22 cells treated for 18 h with the indicated doses of a panel of Flt3 and PI3K inhibitors. (f) Relative survival of HT22 cells stably expressing shRNA targeting Flt3 or PI3Kα and treated with low doses of kinase inhibitors. All survival data are normalized to DMSO control cells incubated without glu or kinase inhibitors. Results are the mean±s.d. ofn=6. In control (dimethyl sulfoxide (DMSO)-treated) cultures, 99% of HT22 cells died, whereas five of the nine tested kinase inhibitors showed varying degrees of protection against glutamate-induced cell death ( Supplementary Table 1 and Fig. 1a ). Figure 1: Kinase inhibitors prevent glutamate-induced cell death. ( a ) Relative HT22 cell survival after treatment with 5 mM glutamate (glu) for 18 h in the presence or absence of the indicated kinase inhibitors (K.I. ; see Supplementary Table 1 ). ( b ) Phase contrast images of HT22 cells treated with 0.5 μM E21 or L13 and 5 mM glu (Scale bar, 50μm). ( c ) Relative cell survival of primary neurons and various neuronal cell lines treated for 18 h with the indicated concentrations of E21 or L13 in the presence of glu at: 5 mM (cerebrocortical neurons, 661W), 10 mM (NSC34) or 20 mM (RGC-5, C6). ( d ) Representative western blots of Flt3, phospho-Flt3, Akt, phospho-Akt and β-actin (control) in lysates of HT22 cells treated with 5 mM glu for 6 h and the indicated concentrations of E21 and L13. ( e ) Relative survival of HT22 cells treated for 18 h with the indicated doses of a panel of Flt3 and PI3K inhibitors. ( f ) Relative survival of HT22 cells stably expressing shRNA targeting Flt3 or PI3Kα and treated with low doses of kinase inhibitors. All survival data are normalized to DMSO control cells incubated without glu or kinase inhibitors. Results are the mean±s.d. of n =6. Full size image The two most effective inhibitors of glutamate-induced death were Flt3 Inhibitor III and PI3Kα Inhibitor VIII (hereafter referred to as E21 and L13, respectively; Supplementary Fig. 1c and Supplementary Table 1 ), which were almost fully protective at doses of 0.5 μM ( Fig. 1a ). HT22 cells exposed to 5 mM glutamate for 18 h lost their normal spindle-shaped morphology, and instead appeared shrunken and rounded, and detached from the culture plate ( Fig. 1b ). In contrast, cells treated with E21 or L13 maintained their normal neurite morphology, similar to cells in DMSO control cultures. We next tested the effect of the inhibitors on glutamate-induced death of primary cerebrocortical neurons and a panel of additional rodent neuronal cells lines. Control cultures of primary neurons displayed normal morphology with short neurites extending to dendritic processes ( Supplementary Fig. 1d ). In contrast, cells exposed to 5 mM glutamate exhibited apoptotic morphology, and this was effectively reversed by co-treatment with either E21 or L13 ( Supplementary Fig. 1d ). We also examined the effect of E21 and L13 on multiple neuronal or neural cell lines known to be susceptible to glutamate-induced toxicity, including 661W (mouse retinal photoreceptor-derived), RGC-5 (rat retinal ganglion) and C6 (rat glioma). Although E21 reproducibly protected all of these cell lines from glutamate-induced death, protection by L13 varied among the cell types, showing excellent activity with C6 cells, for example, and almost no activity with 661W cells ( Fig. 1c ). These compounds were also tested in NSC34 (mouse motor neuron) cells stably expressing a mutant form of superoxide dismutase (SOD), a key antioxidant enzyme. The mutant G93A-hSOD1 gene has been reported to increase cellular oxidative stress, mitochondrial dysfunction and motor neuron cell death [13] . Consistent with this, NSC34 (G93A-hSOD1) cells were more sensitive than wild-type NSC34 cells to the lethal effects of 10 mM glutamate ( Fig. 1c ). However, although E21 was able to prevent NSC34 (G93A-hSOD1) cell death, L13 had the opposite effect, and in this particular case promoted rather than prevented cell death. We next determined the effect of glutamate on endogenous Flt3 and PI3Kα and confirmed the inhibitory effects of E21 and L13. Treatment of HT22 cells with 5 mM glutamate increased the basal level of Flt3 and induced the appearance of the phosphorylated, active forms of Flt3 and the downstream effector of PI3Kα, Akt ( Fig. 1d ). Glutamate-induced phosphorylation of Akt has previously been noted [14] . Both p-Flt3 and p-Akt levels were dose-dependently reduced by the addition of E21 and L13, respectively, demonstrating that both inhibitors effectively block their target kinases following glutamate treatment. To ensure our observations were not limited to E21 and L13, we tested a panel of Flt3 and PI3K inhibitors for their ability to block glutamate-induced death. We found that four of the five Flt3 inhibitors tested were protective to HT22 cells, albeit with differing potencies ( Fig. 1e ). Flt3 Inhibitor I has previously been reported to exhibit poor specificity for Flt3 (ref. 15) [15] , which may explain its inactivity in this assay. Of the panel of PI3K inhibitors tested, protection was observed with all compounds specific for the α isoform but none specific for the PI3Kβ and γ isotypes ( Fig. 1e ). As an additional method of specifically blocking PI3Kα and Flt3 activity, we established HT22 cell lines stably expressing Flt3 or PIK3CA (p110a) shRNA. Silencing of Flt3 and PI3Kα expression synergized with low concentrations of the inhibitors to render the cells more tolerant to oxidative glutamate toxicity, verifying the roles of these kinases in oxidative glutamate toxicity ( Fig. 1f ). Finally, we also tested whether Flt3 ligand could exacerbate glutamate toxicity in HT22 cells, but found no evidence for this ( Supplementary Fig. 1e ), suggesting that Flt3 activity induced by glutamate was sufficient to fully engage cell death pathways. Collectively, these data substantiate the role of Flt3 and PI3Kα in oxidative glutamate toxicity and demonstrated the on-target effects of E21 and L13. Inhibitors prevent ROS production and lipid peroxidation We next determined whether the Flt3 and PI3Kα inhibitors prevented glutamate-induced toxicity in HT22 cells via antioxidant mechanisms. First, intracellular ROS levels were measured by fluorescence-activated cell sorting (FACS) analysis of cells loaded with the cell-permeable fluorogenic probe, 2′,7′-dichlorodihydrofluorescein diacetate (H 2 DCFDA). As previously reported, ROS levels were increased after 6 h of glutamate treatment of HT22 cells compared with untreated cells [6] and that increase was followed by a second burst at 10 h incubation ( Fig. 2a,b ). E21 and L13 effectively prevented both the first and second wave of ROS production, suggesting that their protective activities lie upstream of or at the level of ROS generation ( Fig. 2a,b ). We also confirmed that E21 prevented glutamate-induced ROS production in primary neurons and all of the neuronal cell lines tested, whereas L13 inhibited ROS production only in the cell types in which it prevented cell death ( Fig. 2c ). 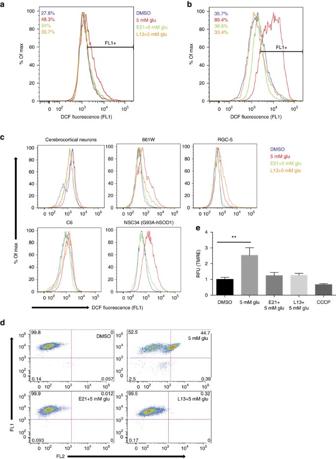Figure 2: Kinase inhibitors prevent ROS production, lipid peroxidation and mitochondrial hyperpolarization induced by glutamate treatment. (a,b) ROS production in HT22 cells assessed by FACS analysis of dichlorofluorescein (DCF) fluorescence (a) 6 h and (b) 10 h after treatment with glu (5 mM)±E21 or L13 (0.5 μM). (c) ROS production by the indicated cells measured 10 h after treatment as in panela. (d) Lipid peroxidation in HT22 cells assessed by FACS analysis of C11-BODIPY fluorescence 8 h after treatment as in panela. (e) Mitochondrial membrane potential measured by relative TMRE fluorescence 8 h after treatment with glu (5 mM)±E21 or L13 (0.5 μM), or with CCCP (50 μM). **P<0.05 (ANOVA). Results are the mean±s.e.m. of three independent experiments. Figure 2: Kinase inhibitors prevent ROS production, lipid peroxidation and mitochondrial hyperpolarization induced by glutamate treatment. ( a,b ) ROS production in HT22 cells assessed by FACS analysis of dichlorofluorescein (DCF) fluorescence ( a ) 6 h and ( b ) 10 h after treatment with glu (5 mM)±E21 or L13 (0.5 μM). (c) ROS production by the indicated cells measured 10 h after treatment as in panel a . ( d ) Lipid peroxidation in HT22 cells assessed by FACS analysis of C11-BODIPY fluorescence 8 h after treatment as in panel a . ( e ) Mitochondrial membrane potential measured by relative TMRE fluorescence 8 h after treatment with glu (5 mM)±E21 or L13 (0.5 μM), or with CCCP (50 μM). ** P <0.05 (ANOVA). Results are the mean±s.e.m. of three independent experiments. Full size image Next, we determined whether Flt3 and PI3Kα inhibition also prevented glutamate-induced lipid peroxidation. Incubation of cells with 5 mM glutamate markedly increased HT22 membrane lipid peroxidation, as measured using the fluorescent dye C11-BODIPY ( Fig. 2d ). Consistent with their observed effects on ROS production, both E21 and L13 prevented this glutamate-induced lipid peroxidation ( Fig. 2d ). Mitochondria can be both a source and a target of ROS-mediated oxidative damage during glutamate toxicity. Mitochondrial membrane function was assessed by uptake of tetramethylrhodamine ethyl ester (TMRE), an indicator of mitochondrial membrane potential. HT22 cells exposed to glutamate showed a relative increase in TMRE fluorescence, indicative of hyperpolarization of the mitochondrial membrane, possibly due to increased ROS production. Consistent with their effects on ROS production and lipid peroxidation, the kinase inhibitors prevented glutamate-induced mitochondrial hyperpolarization whereas carbonyl cyanide m -chlorophenyl hydrazone (CCCP) was used as a control for depolarized mitochondria ( Fig. 2e ). Therefore, we show that mitochondrial hyperpolarization is one of the key functions of glutamate oxidative toxicity and it was prevented by both E21 and L13. Inhibitors block caspase-independent death pathways HT22 cells undergoing glutamate-induced cell death display characteristics of both apoptosis and necrosis [6] , [16] . Although several features of apoptosis, such as cellular condensation and plasma membrane blebbing, occur, DNA fragmentation and chromatin condensation do not. Several studies have suggested that glutamate-induced apoptosis is caspase-independent but AIF-dependent [8] , [17] . We therefore asked whether the Flt3 and PI3Kα inhibitors prevent AIF-mediated execution of caspase-independent apoptotic cell death. Consistent with previous reports, we found that caspases 3/7 were not activated upon glutamate treatment of HT22 cells ( Fig. 3a ), whereas AIF translocated from the mitochondria to the nucleus within 10 h of glutamate treatment ( Fig. 3b ). Notably, E21 inhibited translocation of AIF, whereas L13 could not completely abrogate the process in the presence of 5 mM glutamate ( Fig. 3b ). Thus glutamate-induced death of HT22 cells involves AIF-dependent apoptosis, which is blocked only by Flt3 inhibition. 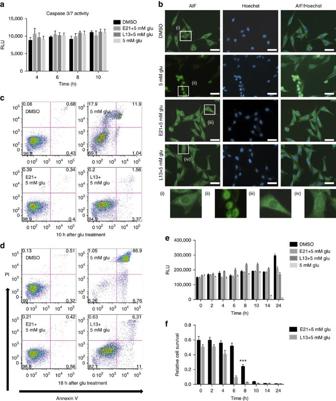Figure 3: Kinase inhibitors reduce glutamate-induced cell death through caspase-independent pathways. (a) Caspase 3/7 activity in HT22 cells 18 h after treatment with glu (5 mM)±E21 or L13 (0.5 μM). (b) Immunostaining of AIF and nuclei (Hoechst) in HT22 cells 10 h after treatment as in panela(Scale bar, 50 μm); (i–iv) show enlarged images of the boxed regions. (c,d) PI/annexin V staining of HT22 cells (c) 10 h and (d) 18 h after treatment as in panela. (e) HT22 cell survival measured at the indicated times after treatment as in panela. (f) HT22 cell survival measured 24 h after incubation with glu (5 mM). L13 or E21 (0.5 μM) were added at the indicated times after addition of glutamate. The 24 h time point shows cell survival after incubation with glu in the absence of inhibitors. The statistical analysis was performed against the values from 24 h time points. ***P<0.001 (ANOVA). Results are the mean±s.d. ofn=6. Figure 3: Kinase inhibitors reduce glutamate-induced cell death through caspase-independent pathways. ( a ) Caspase 3/7 activity in HT22 cells 18 h after treatment with glu (5 mM)±E21 or L13 (0.5 μM). ( b ) Immunostaining of AIF and nuclei (Hoechst) in HT22 cells 10 h after treatment as in panel a (Scale bar, 50 μm); (i–iv) show enlarged images of the boxed regions. ( c , d ) PI/annexin V staining of HT22 cells ( c ) 10 h and ( d ) 18 h after treatment as in panel a . ( e ) HT22 cell survival measured at the indicated times after treatment as in panel a . ( f ) HT22 cell survival measured 24 h after incubation with glu (5 mM). L13 or E21 (0.5 μM) were added at the indicated times after addition of glutamate. The 24 h time point shows cell survival after incubation with glu in the absence of inhibitors. The statistical analysis was performed against the values from 24 h time points. *** P <0.001 (ANOVA). Results are the mean±s.d. of n =6. Full size image Glutamate-treated HT22 cells also show morphological characteristics of necrosis, such as degradation of cytoplasmic organelles and cell swelling [6] . Using propidium iodide (PI)/annexin V staining to discriminate between apoptosis and necrosis, we found that glutamate-induced cell death was predominantly necrotic (PI+/annexin V−) at early times (10 h) after glutamate addition, whereas apoptosis (PI−/annexin V+ to PI+/annexin V+) has a larger role at later time points (18 h), consistent with a previous report [16] ( Fig. 3c,d ). L13 protected cells from early-stage necrosis, but not the later phase of apoptosis. In contrast, E21 effectively prevented both necrotic and apoptotic cell death ( Fig. 3c,d ). Next, we determined the time frame in which the kinase inhibitors act to prevent glutamate-induced death. ATP levels in HT22 cells were measured every 2 h for 24 h. The ATP content of control DMSO-treated cells doubled after 24 h of culture, whereas that of glutamate-treated cells dropped dramatically between 10 and 14 h, consistent with cell death. As expected, cells treated with E21 and L13 maintained their ATP levels at both the 14 and 24 h time points although L13 caused a transient increase in ATP levels between 6 and 10 h during glutamate exposure. ( Fig. 3e and Supplementary Fig. 2 ). Cell survival was then measured after 24 h incubation with glutamate, with the inhibitors added at varying time points between 0 and 14 h. Cultures in which L13 was added after 4 h showed a marked decrease in cell survival at 24 h, indicating that L13 must be present within ~2 h of glutamate addition to prevent cell death ( Fig. 3f ). This is consistent with the results of the PI/Annexin V staining experiments, which showed that L13 mainly protected cells from early necrosis ( Fig. 3c,d ). On the other hand, E21 still showed significant protective activity when added as late as 8 h after the initiation of glutamate exposure. These results suggest that inhibition of PI3Kα kinase activity affects cell death events occurring soon after exposure to glutamate, whereas Flt3 kinase inhibition affects both early and late events in the cell death pathways. Inhibitors prevent ferroptosis and lipid peroxidation Recent studies have described a new, iron-dependent form of cell death, termed ferroptosis [9] . Ferroptosis is distinct from apoptosis and necrosis, but is known to share a common death mechanism with glutamate-induced cell death in rat organotypic hippocampal slice cultures [9] . To determine whether ferroptosis might be involved in glutamate-induced toxicity in HT22 cells, we examined the effects of iron addition and depletion on glutamate-mediated cell death. Treatment of cells with three different exogenous sources of iron (iron chloride hexahydrate, ammonium iron citrate or iron citrate) was found to potentiate glutamate-induced cell death, and conversely, incubation with the iron chelator deferoxamine suppressed cell death ( Fig. 4a,b ). These results suggest that ferroptosis has a role in neuronal cell death mediated by oxidative glutamate toxicity. 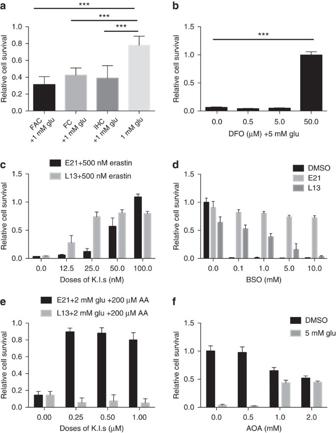Figure 4: Effect of kinase inhibitors on ferroptosis and lipid metabolism. Relative cell survival of HT22 cells 18 h after treatment with (a) glu (1 mM)±10 μg ml−1ammonium iron citrate (FAC), 20 μM iron citrate (FC) or 20 μM iron chloride hexahydrate (IHC); (b) glu (5 mM)±deferoxamine (DFO) at 0.5, 5 or 50 μM; (c) erastin (500 nM)±E21 or L13 at 12.5, 25, 50 or 100 nM; (d) BSO at 0.1, 1, 5 or 10 mM±E21 or L13 (0.5 μM); (e) 2 mM glu plus 200 μM AA±E21 or L13 at 0.25, 0.5 or 1 μM; and (f) glu (5 mM)±AOA at 0.5, 1 or 2 mM. **P<0.05, ***P<0.001 (ANOVA). Results are the mean±s.d. ofn=6. Figure 4: Effect of kinase inhibitors on ferroptosis and lipid metabolism. Relative cell survival of HT22 cells 18 h after treatment with ( a ) glu (1 mM)±10 μg ml −1 ammonium iron citrate (FAC), 20 μM iron citrate (FC) or 20 μM iron chloride hexahydrate (IHC); ( b ) glu (5 mM)±deferoxamine (DFO) at 0.5, 5 or 50 μM; ( c ) erastin (500 nM)±E21 or L13 at 12.5, 25, 50 or 100 nM; ( d ) BSO at 0.1, 1, 5 or 10 mM±E21 or L13 (0.5 μM); ( e ) 2 mM glu plus 200 μM AA±E21 or L13 at 0.25, 0.5 or 1 μM; and ( f ) glu (5 mM)±AOA at 0.5, 1 or 2 mM. ** P <0.05, *** P <0.001 (ANOVA). Results are the mean±s.d. of n =6. Full size image To determine whether E21 and L13 could protect HT22 cells from ferroptotic cell death, HT22 cells were treated with 500 nM erastin, a ferroptosis-inducing agent, with or without L13 or E21 (ref. 18) [18] . Incubation with erastin for 18 h caused cell death in more than 90% of HT22 cultures but this was inhibited in a dose-dependent manner by concomitant incubation with the kinase inhibitors ( Fig. 4c ). We also noted that inhibition of ferroptosis with ferrostatin-1 suppressed glutamate-induced HT22 cell death, suggesting that ferroptosis is a key death mechanism in oxidative glutamate toxicity ( Supplementary Fig. 3a ). As depletion of GSH levels is a major contributor to oxidative glutamate toxicity, we asked whether the protective effects of the kinase inhibitors might be mediated through modulation of GSH levels. To test this, we depleted intracellular GSH by inhibiting the GSH synthetic enzyme γ-glutamate-cysteine ligase with L-buthionine sulfoximine (BSO). E21 prevented HT22 cell death regardless of the presence of BSO, indicating that its protective capability does not depend on restoring GSH levels, suggesting it is acting downstream of GSH depletion ( Fig. 4d ). In contrast, BSO decreased in a dose-dependent manner the protective capability of L13 suggesting a requirement for restored GSH levels. PUFAs such as arachidonic acid (AA) and linolenic acid are substrates of lipoxygenases (LOX), which are known to trigger an oxidative cascade in glutamate-induced death of HT22 cells [17] . LOX oxidizes PUFAs to their hydroperoxyl intermediates, including hydroperoxyeicosantetraenoic acid in the case of AA [19] . Intrigued by our finding that lipid peroxidation and ferroptosis were prevented by the kinase inhibitors, we sought to determine whether AA metabolism might contribute to these pathways. First, we measured survival of HT22 cells after 18 h incubation with low concentrations of glutamate (1 and 2 mM) or erastin (25 and 50 nM) in the presence or absence of AA. We found that AA significantly potentiated glutamate- and erastin-induced cell death in a dose-dependent manner ( Supplementary Fig. 3b,c ). E21 rescued the cells from AA potentiated death in the presence of glutamate or erastin, whereas L13 was completely ineffective ( Fig. 4e and Supplementary Fig. 3d,e ). Taken together, these results indicate that lipid peroxidation is a key event in glutamate-induced toxicity in HT22 cells and E21, in contrast to L13, acts on the lipid metabolism cascade to block glutamate-mediated toxicity. Fatty acid synthesis partly relies on reductive metabolism of glutamate-derived α-ketoglutarate [20] , [21] . Therefore, we asked whether inhibiting entry of glutamate into the tricarboxylic acid (TCA) cycle would affect glutamate-mediated toxicity. Cells were treated with aminooxyacetic acid (AOA) to inhibit the transaminases that convert glutamate into α-ketoglutarate [22] . We observed that AOA (1–2 mM) rescued HT22 cells from glutamate-mediated cell death suggesting that either glutamate may contribute to the synthesis of lipids that eventually promote glutamate-induced cell death or TCA activity might directly contribute to ROS generation ( Fig. 4f ). 1 H-NMR profiling reveals distinct effects of inhibitors Next, we used a 1 H-NMR metabolomics approach to characterize the metabolic changes involved in oxidative glutamate toxicity. Multivariate statistical modelling using principal component analysis (PCA) was performed on the 1 H-NMR spectra of polar fractions of HT22 cells incubated with 5 mM glutamate with or without E21 or L13, or control DMSO-treated cells. The score plots from PCA (PC1 versus PC2) revealed clear separations between the intracellular metabolomes of the control (DMSO) and glutamate-treated cells, with greater separation at the 8 h than the 4 h time point ( Fig. 5a ). Interestingly, PCA scores of L13-treated cells showed very distinct separation from those of cells treated with DMSO or glutamate alone, suggesting that L13 affects intracellular metabolism in a distinctive manner. The loading plots on PC1 were analysed further to obtain a more detailed view of the intracellular metabolites. Expanded sections (2.2–2.5 and 2.78–3 p.p.m.) of the averaged 1 H-NMR spectra for each treatment group are shown in Fig. 5b . One metabolite significantly affected by L13 was GSH, which was significantly reduced by glutamate treatment but also significantly rescued by the addition of L13 ( Fig. 5b,c ). In addition, the total amount of GSH+oxidized GSH was completely depleted at 8 h with glutamate treatment but was partially and significantly restored by the addition L13 but not E21 ( Fig. 5c ). These observations are in line with our finding that L13 is less effective in rescuing cell death by BSO-induced GSH depletion ( Fig. 4d ). Unexpectedly, we found that L13 treatment induced the accumulation of several free amino acids, including Asp, Ala, Gln, Ile, Leu, Pro, Ser, Thr and Val ( Fig. 5d ). In particular, the amino acids synthesized from glutamate, Gln and Pro, were among those significantly elevated. We also noted a decrease in phosphocholine and increase in glycero-3-phosphocholine levels in cells treated with the PI3Kα inhibitor, which is in agreement with published studies ( Supplementary Fig. 4 ) [23] , [24] . 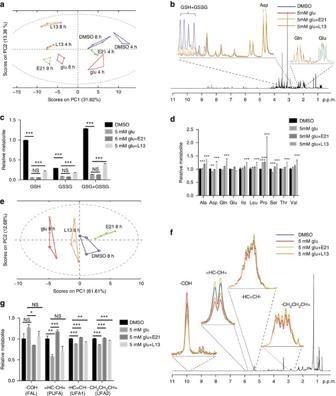Figure 5:Metabolic analyses of the effects of glutamate and kinase inhibitors on polar and apolar fractions of HT22 cells using1H-NMR. (a) PCA score plot for the polar fractions of HT22 cells treated with glu (5 mM)±E21 or L13 (0.5 μM) for 4 or 8 h. (b) Expanded sections of loading plots (right2.2–2.5 andleft2.78–3.0 p.p.m.) of the polar metabolic fractions from cells 8 h after treatment. (c,d) Relative quantification of (c) reduced and oxidized GSH and (d) amino acids in HT22 cells 8 h after treatment. (e) PCA score plot for the lipid fraction of HT22 cells treated with glu (5 mM)±E21 or L13 (0.5 μM) for 8 h. (f) Expanded sections of loading plots of the lipid metabolic fractions. (g) Relative quantification of lipid metabolites. **P<0.05, ***P<0.001, NS=not significant (ANOVA). Data are the mean±s.e.m. from four independent experiments and the statistical analysis was performed against the values from DMSO control cultures. Figure 5: Metabolic analyses of the effects of glutamate and kinase inhibitors on polar and apolar fractions of HT22 cells using 1 H-NMR. ( a ) PCA score plot for the polar fractions of HT22 cells treated with glu (5 mM)±E21 or L13 (0.5 μM) for 4 or 8 h. ( b ) Expanded sections of loading plots ( right 2.2–2.5 and left 2.78–3.0 p.p.m.) of the polar metabolic fractions from cells 8 h after treatment. ( c , d ) Relative quantification of ( c ) reduced and oxidized GSH and ( d ) amino acids in HT22 cells 8 h after treatment. ( e ) PCA score plot for the lipid fraction of HT22 cells treated with glu (5 mM)±E21 or L13 (0.5 μM) for 8 h. ( f ) Expanded sections of loading plots of the lipid metabolic fractions. ( g ) Relative quantification of lipid metabolites. ** P <0.05, *** P <0.001, NS=not significant (ANOVA). Data are the mean±s.e.m. from four independent experiments and the statistical analysis was performed against the values from DMSO control cultures. Full size image We next analysed the 1 H-NMR spectra of the lipid fraction for each treatment group. The score plots from PC1 and PC2 of the lipid fraction showed excellent separation between groups treated with DMSO and glutamate alone ( Fig. 5e ), and the group treated with E21 clustered closer to the DMSO group than to the glutamate control group. Notably, E21 reversed the glutamate-induced changes in lipid metabolism. For example, the levels of free PUFAs were decreased on treatment with glutamate but were completely restored by E21 treatment ( Fig. 5f,g ). Conversely, fatty acid aldehyde products, which were increased after glutamate treatment, were reduced in cells treated with E21 ( Fig. 5f,g ). In HT22 cells, an in vitro model system devoid of N-methyl- D -aspartate receptors, glutamate triggers cell death via oxidative stress resulting from inhibition of cystine uptake and subsequent depletion of GSH [3] , [25] . The present study shows that Flt3 and PI3Kα inhibitors prevent oxidative glutamate toxicity in multiple neuronal cell lines and primary cerebrocortical neurons. Although many inhibitors have been shown to protect neuronal cells from oxidative toxicity [14] , [26] , [27] , [28] , our study not only describes novel effective inhibitors, but also provides new insights into the death mechanisms triggered by oxidative glutamate toxicity. Considerable controversy exists regarding the death mechanisms induced by glutamate oxidative stress. The general view is that oxidative glutamate toxicity triggers necrosis as well as caspase-independent but AIF-dependent apoptosis [6] , [16] , [17] . Previous studies suggested that necrotic cell death is induced early after glutamate treatment (8–12 h), whereas apoptosis is induced at later time (16–24 h) [16] . Our results also showed predominantly necrotic cell death at early time points, which was inhibited by both Flt3 and PI3Kα inhibitors, whereas the later phase of apoptosis was inhibited only by the Flt3 inhibitor. ROS formation and mitochondrial dysfunction are key characteristics of oxidative glutamate toxicity. Our finding that a PI3Kα inhibitor inhibits ROS production suggested a close relationship between ROS production and necrotic cell death. Nec-1, a necrosis inhibitor, has been reported to inhibit glutamate-induced cell death by decreasing ROS production, consistent with a role for necrosis in oxidative glutamate toxicity [7] . However, in that study, Nec-1 also blocked translocation of mitochondrial AIF, an apoptotic event, indicating that necrosis and apoptosis are not completely independent mechanisms in oxidative glutamate toxicity. In our study, the Flt3 inhibitor impeded both glutamate-mediated apoptosis and necrosis. The compound inhibited AIF translocation from the mitochondria to the nucleus, an event occurring downstream of 12, 15-LOX activation. In the model of glutamate oxytosis, GSH depletion leads to lipid peroxidation through activation of 12, 15-LOX, which leads to mitochondrial damage and subsequent release of mitochondrial AIF to the nucleus, triggering apoptosis [8] , [17] , [29] . We showed that this cascade of apoptotic events was completely prevented by inhibition of Flt3 but not by inhibition of PI3Kα. It is interesting to note that the Flt3 inhibitor also acts upstream of this death cascade at the level of lipid metabolism. Lipid metabolism has an important role in oxidative glutamate toxicity, and a prominent role for 12, 15-LOX in ROS production has been previously reported [17] , [29] . LOX oxidizes PUFAs such as AA and linolenic acid into lipid hydroperoxides, subsequently leading to the production of multiple aldehydes, including 4-hydroxynonenal. Therefore, PUFAs are predicted to decrease when lipid peroxidation is increased. Consistent with this, 1 H-NMR analysis showed decreased PUFAs and increased multiple aldehydes after glutamate addition; events that were completely inhibited by the Flt3 inhibitor. Interestingly, several studies have detected increased lipid peroxidation with decreased PUFAs and increased 4-hydroxynonenal in the amygdala and hippocampus of Alzheimer’s disease brain [30] , [31] . Similar patterns of PUFA metabolism were also reported in substantia nigra of Parkinson’s disease brain [32] . Our finding that AA exacerbates glutamate-induced toxicity and that Flt3 inhibition prevents this is also in line with the restoration of PUFA levels by the Flt3 inhibitor in glutamate-stimulated cultures. Together, these observations suggest that Flt3 inhibitors could be a pharmacological candidate for treatment of Alzheimer’s and Parkinson’s diseases and other neurodegenerative disease models where oxidative stress plays a pathogenic role. Another interesting finding in our study is that the death pathway induced by glutamate oxidative stress involves ferroptosis, a newly established iron-dependent death mechanism [9] . Ferroptotic cell death is characterized by the accumulation of lethal levels of lipid ROS. It is plausible that iron catalyses free radical reactions leading to lipid peroxidation, which is inhibited by iron-chelating agents. In the present study, glutamate toxicity in HT22 cells was suppressed by ferrostatin-1, an inhibitor of ferroptosis, whereas the addition of iron-amplified glutamate-induced cell death, substantiating a role for iron in glutamate oxytosis. Moreover, both kinase inhibitors also protected HT22 cells from erastin-induced ferroptosis. It is notable that AA potentiated erastin-induced ferroptosis, implying an association between ROS production and PUFAs in ferroptosis. To our knowledge, this is the first demonstration of the involvement of PUFA metabolism in ferroptosis. Our results show that glutamate toxicity was attenuated when glutamate entry into the TCA cycle was blocked by AOA, a transaminase inhibitor. One possible explanation for this effect is that import of glutamate into the TCA cycle via α-ketoglutarate contributes to elevated oxidative phosphorylation, subsequent ROS production, and oxidative stress. In fact, we showed that glutamate treatment induces mitochondrial hyperpolarization that is abolished by the addition of PI3Kα and Flt3 inhibitors. The importance of mitochondrial respiration in oxidative damage has been reported [33] . It is likely that elevated mitochondrial oxidative phosphorylation produces ROS as undesired byproducts, thus increasing the mitochondrial potential and further amplifying lipid ROS production. Although a few studies have reported mitochondrial depolarization after glutamate treatment in HT22 cells, the experiments were performed at later time points when the cells were already dying [8] , [34] . We noted changes in mitochondrial potential at 8 h after glutamate treatment, which coincided with the time points of lipid peroxidation and the second ROS burst, thus indicating a close association between mitochondrial damage and ROS production. Our results are supported by a recent study showing that glutamate-induced cytotoxicity is associated with mitochondrial hyperpolarization and increased ROS production [35] . It is also possible that glutamate may contribute to the synthesis of lipids that eventually promote glutamate-induced cell death. Our results with the PI3Kα inhibitor are contrary to the recognized role of PI3K in cell survival. The prosurvival/antiapoptotic functions of PI3K are well established [36] , [37] , [38] , and the PI3K–Akt pathway is known to have an important role in neuronal cell survival [38] . However, evidence also exists that transient inhibition of the PI3K–Akt pathway protects neuronal cells from glutamate-induced oxidative toxicity, suggesting that PI3K may have opposing roles in different cellular contexts [14] , [39] . The role of PI3K implied by our results may be attributed to effects on necrotic death that oppose its prosurvival function (for example, against N-methyl- D -aspartate receptor-mediated apoptotic cell death). Our observation that NSC34 motor neuron cells with mutant G93A-hSOD1 were killed by treatment with L13 provides evidence for the dual functions of PI3Kα pathways. The conflicting reports of the effects of PI3K inhibition may be due to isoform selectivity (see Fig. 1e ). Multiple PI3K isoforms exist, and ensuring isoform selectivity of inhibitors is one challenge of pharmacological target validation. Although Wortmannin and LY294002 are widely employed PI3K inhibitors, they are broadly active within the PI3K family and the reported protective activity of LY294002 ranges from 10 to 30 μM [39] . In contrast, the PI3Kα inhibitor used here shows high specificity for the α isoform, is protective at doses between 0.1 and 1 μM and its target selectivity has been well defined in previous publications [40] , [41] . The importance of selective inhibition of PI3Kα is confirmed by the results with multiple inhibitors shown in Fig. 1e . Although PI3Kγ has recently been reported to contribute to glutamate-induced H 2 O 2 generation [14] , our study instead shows a role for PI3Kα in glutamate oxidative toxicity. We found that the PI3Kα inhibitor can restore GSH levels in HT22 cells. In non-neuronal cells, oxidative stress has been shown to increase PI3K activity, and PI3K inhibition decreases ROS levels and oxidative stress-induced calcium release [42] , [43] , [44] . These earlier observations might be explained by our demonstration of the role of PI3Kα inhibition in restoration of GSH levels. Activation of Akt, which is directly downstream of PI3Kα, can both induce ROS-mediated cell death and inhibit apoptosis, suggesting that the dual modes of action of PI3K/Akt in cell death/survival involve ROS [45] . Our initial screen identified five kinase inhibitors of which Flt3 Inhibitor III (E21) and PI3Kα Inhibitor VIII (L13) were selected based on their potencies. It should be noted, however, that the other three candidate inhibitors are also Flt3 inhibitors, either specifically (E9; Supplementary Table 1 ) or as one of several targets (C16 and O20) [15] , [46] . In addition, a panel of Flt3 inhibitors (including E21, Flt3 inhibitor II, Flt3 inhibitor IV and Quizartinib, an FDA approved drug) showed protective capability against glutamate oxytoxicity (see Fig. 1e ). Flt3 Inhibitor III (E21) shows minimal off-target interactions with high-target selectivity [15] and its efficacy was shown in multiple cell lines and in primary neurons ( Fig. 1c ). This, together with the results of shRNA-knockdown experiments, confirms that the protective action of E21 is mediated by inhibition of the catalytic activity of Flt3. Although numerous studies have investigated the function of Flt3 during hematopoiesis, few studies have focused on its role in neuronal cells [47] . A few studies in cancer models have reported that activating mutations of Flt3 increase ROS levels, and this was blocked by Flt3 inhibition [48] , [49] . Consistent with these reports, we demonstrated a role for Flt3 inhibition in the suppression of lipid peroxidation and ROS production. Constitutive activation of Flt3 triggers a number of distinct downstream pathways, including PI3K/Akt, Ras/MEK/MAPK and STAT [50] . There is some evidence [48] , [49] , [50] , [51] , [52] that these downstream targets have a role in ROS production, thereby linking inhibition of upstream Flt3 to the prevention of ROS-mediated cell death. Sallmyr et al. [48] have reported STAT5 signalling as a possible mechanism leading to ROS generation; they found that STAT5 activates RAC1, which is required to bind NADPH oxidase for ROS production. Another downstream target of Flt3, Ras, was also reported to upregulate ROS levels [51] and increase 5-LOX [52] and 12-lipoxygenase activities [53] . In summary, our study demonstrated the protective roles of Flt3 and PI3Kα inhibitors against glutamate-induced oxidative stress and further elucidated the death mechanisms triggered by glutamate, proving the involvement of lipid peroxidation-mediated ferroptosis as well as necrosis and apoptosis in glutamate oxytosis ( Fig. 6 ). The protective effect of Flt3 inhibitors was more general as it was confirmed in more cell types than the effect of the PI3Kα inhibitors, which in some cases had cytotoxic effects. We propose that Flt3 inhibitors, and to a lesser extent PI3Kα inhibitors, may be useful for understanding and treating neuronal diseases associated with oxidative stress, particularly lipid radical-mediated oxidative toxicity. These inhibitors may thus potentially be relevant to devise future treatments, such as combination therapies, for ischaemic stroke, amyotrophic lateral sclerosis, Parkinson’s disease and Alzheimer’s disease. 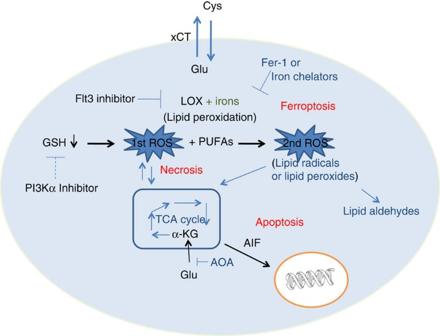Figure 6: Proposed mechanisms of glutamate-induced death in HT22 cells. Based on the results presented here, we propose a model in which glutamate induces GSH depletion and mitochondrial hyperactivation via increased TCA cycle activity, which elevates ROS levels and causes necrotic cell death. ROS production can facilitate lipid peroxidation catalysed by iron, leading to a second burst of ROS production and ferroptotic cell death. The second wave of ROS production further damages the mitochondria and triggers apoptosis accompanied by the translocation of AIF from damaged mitochondria to the nucleus. Flt3 inhibitors are proposed to prevent ROS production, lipid peroxidation and subsequent death cascades, whereas PI3Kα inhibitors are proposed to block the initial wave of ROS production by partially restoring depleted GSH levels. Figure 6: Proposed mechanisms of glutamate-induced death in HT22 cells. Based on the results presented here, we propose a model in which glutamate induces GSH depletion and mitochondrial hyperactivation via increased TCA cycle activity, which elevates ROS levels and causes necrotic cell death. ROS production can facilitate lipid peroxidation catalysed by iron, leading to a second burst of ROS production and ferroptotic cell death. The second wave of ROS production further damages the mitochondria and triggers apoptosis accompanied by the translocation of AIF from damaged mitochondria to the nucleus. Flt3 inhibitors are proposed to prevent ROS production, lipid peroxidation and subsequent death cascades, whereas PI3Kα inhibitors are proposed to block the initial wave of ROS production by partially restoring depleted GSH levels. Full size image Chemicals The following chemicals were purchased from Sigma Aldrich: iron chloride hexahydrate, iron citrate, ammonium iron citrate, deferoxamine mesylate salt, erastin L-glutamate, AA, AOA, hydrogen peroxide and CCCP. The EMD kinase library, PI3Kγ /CKII Inhibitor, PI3Kβ Inhibitor VI, PI3Kγ Inhibitor VII, PI3Kα Inhibitor IV, PI3Kα Inhibitor VIII and Flt3 Inhibitors I, II, III were purchased from EMD Bioscience. GDC0032 and BYL-719 were purchased from Active Biochem. Quizartinib was purchased from Selleckchem. Cell culture and cell survival assays The mouse and rat neuronal cells lines HT22 (a gift from Dr Takumi Satoh), 661W (a gift from Dr Stuart Lipton), RGC-5 (a gift from Dr Won-kyu Ju) and C6 (a gift from Dr Minoru Fukuda) were maintained in Dulbecco’s modified Eagle’s medium (DMEM, Invitrogen) supplemented with 10% fetal bovine serum (FBS, Hyclone), 100 U ml −1 penicillin, and 100 μg ml −1 streptomycin (Hyclone) at 37 °C in a humidified 5% CO 2 atmosphere. Mouse NSC34 cells stably transfected with G93A-hSOD1 or empty vector (gifts from Dr Nick Cosford) were cultured in DMEM supplemented with 10% FBS, 100 U ml −1 penicillin, 100 μg ml −1 streptomycin, 25 mM HEPES, and were selected in medium containing 500 μg ml −1 of G418 (Invitrogen). Cell survival was quantified with the luciferase-based assay, ATPlite (PerkinElmer), which measures ATP levels in metabolically active cells. Cells were seeded overnight at 10 3 or 5 × 10 3 cells per well (for 384- or 96-well plates, respectively). Compounds or DMSO were added the next day and the cells were cultured for 18 h before the ATPlite assay was performed according to the manufacturer’s protocol. Luminescence was read with an Analyst HT apparatus (Molecular Devices). Results are representative of at least three independent experiments each with six replicates. For experiments with amino acid-deficient media, cells were seeded in cystine- and methionine-free DMEM (Invitrogen) supplemented with or without 10% dialysed FBS, 100 U ml −1 penicillin and 100 μg ml −1 streptomycin. Primary cerebrocortical cell culture Rat primary cortical neurons were isolated from cerebral cortexes of Sprague–Dawley rat fetuses on E16, as described by Medders et al. [54] Briefly, whole cerebral neocortices were removed from the rat fetuses, and incubated in 0.03% trypsin in Earle’s balanced salt solution (EBSS) without Ca 2+ or Mg 2+ for 90 min at 37 °C. Subsequently, the cortices washed with fresh Earle’s balanced salt solution, transferred into culture medium (12.5% F-12 growth media (Sigma), 12.5% heat-inactivated horse serum (Hyclone), 30 U ml −1 penicillin, 0.03 mg ml −1 streptomycin solution (both Sigma), 2.5 mM glutamine (Sigma), 10 mM HEPES (Omega) in DMEM with high glucose (4,500 g l −1 , Sigma) and dissociated by trituration. Cells were seeded in poly-D-lysine-treated 384-well culture plates at a density of 5 × 10 4 cells per well and cultured for 2 to 3 days at 37 °C in a 7.5% CO 2 atmosphere before the glutamate exposure experiments. EMD library screen The EMD kinase inhibitor library was screened for the ability to protect cells from hypoxia-induced cell death. Cells were plated at 10 3 cells per well in 384-well plates in DMEM containing DMSO or library compounds at 1 μM final concentration. Cells were cultured in an airtight modular hypoxia chamber under 0.1% hypoxic conditions for 72 h, and the ATPlite cell survival assay was then performed. Relative cell-survival values from quadruplicate wells were averaged and rank ordered from the highest to the lowest cell survival. Using a cut-off value of at least 30% increase in cell survival compared with control DMSO-treated cells, the nine most effective kinase inhibitors were selected for testing in full dose-response curves to confirm their activity. Analysis of oxidative stress Quantification of intracellular ROS was performed with H 2 DCFDA, a non-fluorescent dye, which is converted to the highly fluorescent dichlorofluorescein on oxidation by intracellular ROS. Cells were subjected to experimental treatments and then incubated with 10 μM H 2 DCFDA (Invitrogen) for 30 min. Cell fluorescence was immediately analysed by FACS using a FACSCanto flow cytometer (BD Biosciences) at an excitation wavelength of 488 nm. For detection of cellular lipid peroxidation, cells were treated experimentally and then loaded with 1 μM BODIPY 581/591 C11 (Invitrogen) for 1 h. Cells were collected and analysed by FACS at 530 and 585 nm. A minimum of 10,000 events per replicate was collected and the results are representative of three independent experiments. FACS data were subsequently analysed with FlowJo software (TreeStar). FACS analysis of apoptotic and necrotic cell death Apoptotic and necrotic cell death were detected by staining with PI and annexin V. Cells were collected, resuspended in buffer containing fluorescein isothiocyanate-conjugated annexin V and PI (BD Biosciences) for 15 min at room temperature, and immediately analysed by FACS. A minimum of 10,000 events was collected per sample. shRNA transfection Flt3, PIK3CA and control (scrambled) shRNAs (Target sequences of Flt3: CGCTAACTTCTATAAACTGAT, GCAGGAGAATACCTACTCCAT and PIK3CA: CGAATCCTAGTGGAATGTTTA, GCCTTTCAATCTGCTCTGTTA) were purchased from Thermo Scientific (TRC-pLKO.1 bacterial glycerol stock). Lentiviral shRNA clones were packaged in HEK293T cells and harvested lentiviruses were used for infection of HT22 cells. HT22 cells stably expressing shRNAs were selected by passaging in puromycin-containing media. The knockdown efficiency was confirmed by immunoblot analysis ( Fig. 1f ). Immunoblotting Cells were either lysed in ice-cold radioimmunoprecipitation assay buffer containing a protease inhibitor cocktail or resuspended directly in SDS–PAGE sample buffer. After SDS–PAGE and protein transfer, blots were incubated with primary antibodies to Flt3 (1:1,000), phospho (p)-Flt3 (Tyr 589/591) (1:1,000), Akt (1:1,000) or p-Akt (Ser 473; 1:500; all from Cell Signalling Technology) overnight at 4 °C followed by incubation with horseradish peroxidase-conjugated secondary antibodies at room temperature. Protein bands were detected with ECL detection reagent (GE Healthcare). Blots were probed with an anti-β-actin antibody (1:1,000; Cell Signalling Technology) as a loading control. Whole blot images are presented in Supplementary Fig. 5 . Measurement of mitochondrial membrane potential Quantitation of mitochondrial membrane potential in live cells was performed with TMRE. After experimental treatment, cells were labelled with 250 nM TMRE (Invitrogen) for 20 min at 37 °C, and then harvested by trypsinization and resuspended in 150 nM TMRE. Cells were analysed immediately by FACS. As positive control for depolarization, 50 μM CCCP was applied to cells 1 h before TMRE labelling. Detection of caspase-3,7 activity and cell cytotoxicity Caspase-3 and -7 activities were measured using a luminescence-based assay, Caspase-Glo 3/7 Assay (Promega), according to the manufacturer’s protocol. In brief, cells were incubated with substrate (Ac-DEVD-pNA) for 30 min at room temperature and luminescence was measured with an Analyst HT apparatus. Cytotoxicity was assessed with CytoTox-Fluor Cytotoxicity Assay (Promega), a fluorescence-based assay that uses a fluorogenic peptide substrate (bis-alanyl-alanyl-phenylalanyl-rhodamine 110; bis-AAF-R110) to quantify protease activity released from dead cells. The relative number of dead cells was measured by measuring fluorescence at 485 nm (excitation) and 520 nm (emission). Immunocytochemistry For immunohistochemical detection of AIF, cells were fixed in 4% paraformaldehyde in phosphate-buffered saline (PBS) for 20 min at room temperature and then permeabilized in 0.2% Triton X-100/PBS for a further 20 min. Cells were blocked by incubation with 3% bovine serum albumin (BSA) in PBS, incubated with goat anti-AIF (1:200 dilution; Santa Cruz Biotechnology) overnight at 4 °C, and then incubated with Alexa 488-labelled donkey anti-goat secondary antibody (1:400; Invitrogen) for 1 h at room temperature. Cells were counterstained with Hoechst 33342 (Invitrogen) to visualize nuclei. NMR analysis For NMR sample preparation, 7 × 10 6 HT22 cells were incubated for 4 or 8 h, harvested in ice-cold methanol and snap-frozen immediately. Four replicate samples were collected per treatment. Extraction of intracellular metabolites was performed as described previously [55] . One dimensional standard 1 H-NMR data were acquired on 700-MHz Bruker and 600-MHz Bruker Avance spectrometers equipped with a TCI cryoprobe (Bruker BioSpin Corp., MA, USA). The acquisition parameters for 1D spectra were a 90° flip angle, 6 kHz spectral width, relaxation delay of 1 s, 16,000 data points and 8 dummy scans. Carr–Purcell–Meiboom–Gill 1 H spectra for lipid fractions were recorded using spin–spin relaxation delay of 100 ms. NMR data were processed using MetaboLab in the MATLAB programming environment (MathWorks Inc., MA, USA) [56] . Post-processing of 1D MRS spectra for the multivariate analysis included scaling according to the probabilistic quotient method, alignment, exclusion of selected signals arising from solvents, trimethylsilyl propanoic acid binning at 0.005 p.p.m. and application of generalized log transformation. Statistical analysis Statistical analyses were performed using Graph Pad Prism (GraphPad Software, CA, USA). Differences between the treatment groups were analysed by two-way or one-way analysis of variance (ANOVA) with Sidak correction for multiple comparisons. How to cite this article: Kang, Y. et al. Cellular protection using Flt3 and PI3Kα inhibitors demonstrates multiple mechanisms of oxidative glutamate toxicity. Nat. Commun. 5:3672 doi: 10.1038/ncomms4672 (2014).